Biologically inspired pteridine redox centres for rechargeable batteries The use of biologically occurring redox centres holds a great potential in designing sustainable energy storage systems. Yet, to become practically feasible, it is critical to explore optimization strategies of biological redox compounds, along with in-depth studies regarding their underlying energy storage mechanisms. Here we report a molecular simplification strategy to tailor the redox unit of pteridine derivatives, which are essential components of ubiquitous electron transfer proteins in nature. We first apply pteridine systems of alloxazinic structure in lithium/sodium rechargeable batteries and unveil their reversible tautomerism during energy storage. Through the molecular tailoring, the pteridine electrodes can show outstanding performance, delivering 533 Wh kg −1 within 1 h and 348 Wh kg −1 within 1 min, as well as high cyclability retaining 96% of the initial capacity after 500 cycles at 10 A g −1 . Our strategy combined with experimental and theoretical studies suggests guidance for the rational design of organic redox centres. Organic materials represent an attractive alternative to transition metal oxide cathodes in conventional rechargeable batteries because of their light weight, structural flexibility and chemical diversity [1] , [2] . In particular, organic molecules that mimic redox centres in biological energy transduction have gained a great deal of attention for their sustainability and universal availability in natural systems [3] , [4] . For instance, carbonyl-based compounds are the most well-known examples of bio-inspired redox centres, imitating quinone cofactors in nature, such as plastoquinone and ubiquinone, which are involved in the electron transport chain of chloroplasts and mitochondria [5] , [6] , [7] , [8] , [9] . Previous studies on these compounds have shown promising electrochemical properties with high energy densities [10] , [11] , [12] , [13] . Recent efforts have enabled the carbonyl-based organic electrodes to have high power as well as stable cycling performance, hinting at a practical feasibility for a bio-inspired design of energy storage materials [10] , [14] , [15] , [16] , [17] . As a wide range of ion-coupled electron transfer reactions exists in biological energy conversion, the characterization of these redox systems may provide novel methods of electrochemical energy storage with versatile functionalities. In living organisms, heterocyclic molecules containing a pteridine (1,3,5,8-tetraazanaphthalene) nucleus composed of fused pyrimidine and pyrazine rings are widely occurring redox centres [18] , [19] . Among such molecules, flavin cofactors including FAD and flavin mononucleotide are one of the most vital compounds that catalyse biotransformation and energy transfer reactions [20] . During photosynthesis and cellular respiration, for example, flavin cofactors serve as a key redox centre facilitating proton-coupled electron transfer reactions for energy transduction. During the reaction, redox cycling occurs at the diazabutadiene of the isoalloxazine moiety [21] , [22] . On the basis of this electrochemical cellular metabolism, we recently proposed that natural flavin cofactors can be applied to lithium-storing electrodes in rechargeable batteries [23] . Although flavin-based electrodes can reversibly facilitate lithium-coupled electron transfer in batteries, their inadequate performance in terms of energy density and cycle stability requires further optimization along with in-depth studies regarding the underlying energy storage mechanism in the battery systems. In this report, we present a molecular simplification strategy to design a minimal redox-active unit of the diazabutadiene redox cycle using chemical tailoring. The resulting pteridine derivatives in the alloxazinic structure are first used in lithium and sodium rechargeable battery systems as a novel class of organic cathodes. Spectroscopic and computational studies reveal differences in the underlying energy storage mechanisms between pristine isoalloxazic and derived alloxazinic systems. Furthermore, by introducing nanocarbons as a conductive scaffold for molecule immobilization during electrode preparation, we demonstrate that the pteridine derivatives exhibit outstanding electrochemical performance in terms of power and cyclability in battery operations. Molecular tailoring of pteridine systems for energy storage To increase energy density, we simplified the chemical structure of flavin molecules by removing non-redox-active substituents from the molecules while maintaining the redox-active moiety ( Fig. 1a ). The centre of redox reactivity in flavins is the isoalloxazine ring system, specifically the conjugated diazabutadiene (N5-C4a-C10a-Ni1) region that facilitates the lithium-coupled electron transfer reaction via sequential reduction of N5 and N1 ( Fig. 1b ) [23] . Without the ribityl substituents, which yields a simpler molecule lumichrome (7,8-dimethylalloxazine, LC), flavin could no longer maintain its isoalloxazinic form. Rather, LC formed an alloxazinic structure, in which N1 and N3 (instead of N10 and N3) are substituted as shown in Fig. 1a (ref. 24 ). Although the structures of isoalloxazinic and alloxazinic molecules are closely related, the chemical and physical properties of these two systems differ significantly [25] . For example, each system shows different photoemission bands: the excited-state lifetime of the isoalloxazinic structure is longer than that of the alloxazinic structure, and the isoalloxazinic structure exhibits stronger emission intensity. On the basis of these photophysical differences, previous studies on LC observed an interesting phenomenon called excited-state tautomerism, which is a structural isomerism from the alloxazinic to the isoalloxazinic type ( Fig. 1c ) [26] , [27] . However, few studies have explored the redox chemistry of LC. To the best of our knowledge, the reversible tautomeric reaction of LC during electrochemical reactions has not been demonstrated previously, which will be discussed below. We further searched for simpler forms of the pteridine redox centre by sequentially removing substituents, which are alloxazine (ALX, without the methyl groups at C7 and C8 of LC) and lumazine (LMZ, without the anellated benzo ring of ALX). 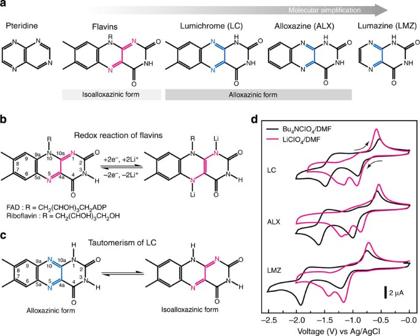Figure 1: Biologically inspired pteridine redox cofactors. (a) Molecular structures of pteridine derivatives as bioinpsired redox compounds for energy storage. (b) Redox mechanism of flavins inspired by biological energy transduction. (c) Reversible tautomerism of LC, which is a structural isomerism from the alloxazinc to the isoalloxazinic type. (d) Cyclic voltammograms of pteridine derivatives measured in DMF solutions containing TBAP (black) and LiClO4(red) as electrolytes. Figure 1: Biologically inspired pteridine redox cofactors. ( a ) Molecular structures of pteridine derivatives as bioinpsired redox compounds for energy storage. ( b ) Redox mechanism of flavins inspired by biological energy transduction. ( c ) Reversible tautomerism of LC, which is a structural isomerism from the alloxazinc to the isoalloxazinic type. ( d ) Cyclic voltammograms of pteridine derivatives measured in DMF solutions containing TBAP (black) and LiClO 4 (red) as electrolytes. Full size image The redox properties of pteridine derivatives were first investigated with cyclic voltammetry using percholate electolytes in N,N-dimethylformamide (DMF) under N 2 atmosphere ( Fig. 1d ). In tetrabutylammonium perchlorate (TBAP), which contains TBA + as noninteracting cations, pteridine derivatives exhibited two reduction and oxidation peaks in the cyclic voltammetry curves. The use of LiClO 4 as a supporting electrolyte resulted in more complicated redox behaviour with positive shifts of the average redox potentials, which is attributed to the possible existence of interacting Li + cation [16] , [28] . Lithium storage mechanism of LC As the first step to utilize pteridine derivatives in lithium storage, we examined the electrochemical activity of the LC electrode versus lithium counter electrode in a coin-type cell. According to our galvanostatic measurements, LC/Li cells could reversibly take up and release two lithium ions and electrons. The specific capacity of LC/Li cell was ~169 mAh g −1 , equivalent to 1.53 Li atoms per molecule between 1.5 and 3.6 V at a current density of 20.0 mA g −1 ( Fig. 2a ). When we apply high temperature (60 °C) to the battery operation of LC, its capacity reached to 181 mAh g −1 ( Supplementary Fig. 1 ). The theoretical capacity corresponding to two Li atoms in the LC electrode is 221 mAh g −1 . Two sets of distinctive cathodic and anodic peaks were observed with average potentials of 2.50 and 2.35 V based on differential capacity curves ( Fig. 2a , inset). The result indicated that the electrode reaction of LC followed two consecutive lithium insertion reactions with a relatively stable intermediate phase, which resembles the redox chemistry of riboflavins in lithium cells [23] . We also performed a galvanostatic intermittent titration technique (GITT) measurement under an intermittent discharge/charge for 1 h at a low current rate of 10.0 mA g −1 with relaxation periods maintained for 5 h. The GITT result in Fig. 2b shows that the open-circuit voltage (OCV) of LC was nearly unchanged at 2.50 V during the first reduction by lithiation, while the OCV continuously decreased during the second stage of the reduction. During the recharge period, the OCV continuously increased to 2.50 V, and then remained flat until the majority of lithium ions were extracted from LC. The flat potential in the electrochemical profile suggests that lithium insertion followed a two-phase-based reaction in the region, which is known to occur in conventional olivine LiFePO 4 electrodes. 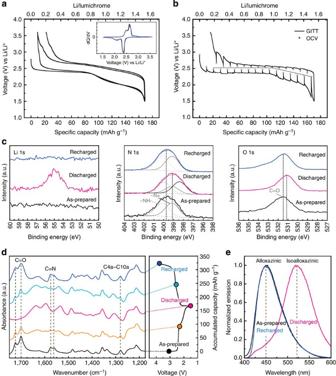Figure 2: Energy storage mechanism of lumichrome. (a) Capacity–voltage profiles and the corresponding differential capacity plots (inset) of LC/Li cells. (b) GITT profiles of the LC/Li cells. (c–e)Ex situanalyses of LC electrodes at different states of charge during battery cycling. (c) XPS local scan spectra of Li 1s, N 1s and O 1s regions, (d) FTIR spectra of CN and CO bonds and (e) emission spectra are reversibly switching on reduction and oxidation of the LC, which is indicative of the redox stability of alloxazinic systems. Figure 2: Energy storage mechanism of lumichrome. ( a ) Capacity–voltage profiles and the corresponding differential capacity plots (inset) of LC/Li cells. ( b ) GITT profiles of the LC/Li cells. ( c – e ) Ex situ analyses of LC electrodes at different states of charge during battery cycling. ( c ) XPS local scan spectra of Li 1s, N 1s and O 1s regions, ( d ) FTIR spectra of CN and CO bonds and ( e ) emission spectra are reversibly switching on reduction and oxidation of the LC, which is indicative of the redox stability of alloxazinic systems. Full size image To characterize the redox mechanism of LC, we performed ex situ experimental and computational studies of the electrode during battery operation. Changes in the crystal structure of LC were first investigated by comparing X-ray diffraction patterns of LC electrodes at various states, including as-prepared, fully discharged and fully recharged states ( Supplementary Fig. 2 ). We found that the as-prepared electrode comprising crystalline LC powders lost the long-range crystalline order on the first discharge and partially restored its original crystallinity on the recharge. The amorphization of the electrodes on cation insertion is often observed for the organic active materials, which is attributable to the relatively weak interactions (van der Waals force, hydrogen bond) among the molecules comprising the crystalline structure [29] , [30] . Nevertheless, the electrodes still retained the redox activity for continuous battery operation, which implies that the electrochemical activities are not dominated by the long-range crystalline order of organic electrode materials. To identify the evolution of molecular structure during the electrochemical reactions, we performed various spectroscopic analyses. High-resolution X-ray photoelectron spectroscopy (XPS) scans of the electrodes confirmed the reversible lithium insertion and extraction in LC during battery cycling ( Fig. 2c ). In the Li 1s spectra, the lithium peaks reversibly evolved with the discharge and disappeared with subsequent charging of the LC electrode. The electron density in nitrogen and oxygen atoms of LC changed according to lithiation and delithiation, suggesting that these atoms are redox-active centres. The peak in the N 1s spectra of the as-prepared electrode (full-width at half-maximum, FWHM: 2.23 eV) was broadened during the discharged state (FWHM: 2.57 eV) and then recovered after recharge (FWHM: 2.25 eV), which shifted the peak to lower energies and then back to the initial value. For the as-prepared electrode, the N 1s spectrum could be deconvoluted into two peaks with the same FWHM of 1.60 eV centred at 399.15 and 400.15 eV, which were assigned to conjugated (sp 2 ) –N= and non-conjugated (sp 3 ) –NH– groups, respectively [31] . After discharge, an additional peak evolved at a lower binding energy, 398.40 eV, while the –N= peak (399.15 eV) decreased, implying that reduction occurred at nitrogen atoms in the pyrazine ring. The new peak could be designated as N–Li, which was similar to that commonly observed in lithium azide [32] . For a recharged electrode, the reversible diminution of the N–Li peak at 398.40 eV, as well as restoration of the –N= peak was observed, which is in agreement with the redox reaction of LC versus lithium. In the O 1s spectra, a slight downshift of the O 1s binding-energy peak was detected in the discharged state, which indicated that the electron density of oxygen atoms also increased during lithiation-involved reduction of LC. Ex situ Fourier transform infrared spectroscopy analysis shown in Fig. 2d further confirmed the reversible change in the molecular structure of LC during the redox reaction involving lithium insertion/extraction. As LC/Li cells were discharged and recharged, peaks at 1,278, 1,561 and 1,578 cm −1 corresponding to the vibrational modes of C4a–C10a single bond and C=N double bonds [33] ( v (N10=C10a), v (N5=C4a)) gradually disappeared and reappeared. This result represents that the conjugated diazabutadiene motif (–N=C–C=N–) participated in the redox reaction of LC, in agreement with the XPS results. In addition, we found that the vibrational modes of C=O bonds [34] were reversibly eliminated and restored not only for C4 but also for C2 at 1,697 and 1,723 cm −1 , respectively, denoting that all lithium insertion reactions occur at the nitrogen atoms neighbouring oxygen atoms. This observation points to an interesting configurational change of the molecule during lithiation. Since N10 does not neighbor a C=O bond, as shown in Fig. 1c , it is expected that the N1 neighbouring C=O participates in lithium accommodation, although the N1 atom is already bound to a proton in the pristine alloxazinic form. This strongly suggests that tautomerism to the isoalloxazinic structure occurred electrochemically to form the N1–Li–O–C2 heterocyclic structure by accompanying proton transfer from N1 to N10. We further monitored the configuration change of LC during reduction and oxidation in battery using fluorescence spectroscopy ( Fig. 2e ). After reduction (that is, discharge), the appearance of isoalloxazinic fluorescence at 520 nm and the disappearance of alloxazinic fluorescence at 450 nm at the discharged state were clearly observed, which agreed with previous reports on phototautomerism [26] , [27] . After recharging, the LC showed fluorescence at 450 nm again, suggesting that the tautomerism of the alloxazinic to the isoalloxazinic structure was completely reversible during the lithium-coupled redox reaction. The photo-induced tautomerism of LC has been well characterized [26] , [27] , but the similar tautomerism to the isoalloxazinic structure that occured electrochemically during lithium-coupled electron reduction was unexpected. Our experimental results on the redox mechanism of LC accompanying tautomerism were supported by density functional theory (DFT) calculations (B3LYP hybrid functional). First, we explored how many electrons could be maximally adopted and how they were distributed in LC by examining the highest occupied molecular orbitals (HOMO) of the molecule. The HOMO plot of a molecule provides qualitative information on its capability of accepting electrons in a given molecular structure [35] . When the LC molecule is reduced by accepting two electrons, effective electron delocalization occurs in the conjugated structure of reduced LC (LC 2− ; Fig. 3a ). Further reduction, however, does not allow the molecule to stabilize the electrons ( Supplementary Fig. 3 ), indicating that LC is capable of a two-electron redox reaction. It was further noted that reduced LC (LC 2− ) was more stable in the isoalloxazinic form than in the pristine alloxazinic form by 0.299 eV. 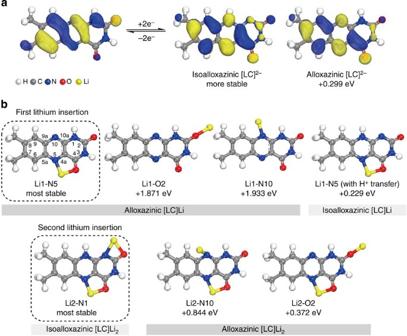Figure 3: DFT calculation on LC during redox reactions. (a) HOMO plots of LC and doubly reduced LC tautomers. (b) DFT energy comparison for various forms of [LC]Li (upper) and [LC]Li2(lower) on two-lithium-coupled two-electron reduction. Figure 3: DFT calculation on LC during redox reactions. ( a ) HOMO plots of LC and doubly reduced LC tautomers. ( b ) DFT energy comparison for various forms of [LC]Li (upper) and [LC]Li 2 (lower) on two-lithium-coupled two-electron reduction. Full size image To improve our understanding on the redox mechanism of LC, we compared DFT energies of possible lithium configurations for [LC]Li and [LC]Li 2 ( Fig. 3b ). It was found that [LC]Li containing N5–Li bond where the lithium ion also interacted with O4 was the most stable structure by more than 1.80 eV among various possible configurations, and the alloxazinic structure was favoured over the isoalloxazinic tautomer by 0.23 eV under vacuum. In a more realistic simulation in the presence of electrolytes, however, we found notable distinction in preferred configuration ( Supplementary Figs 4 and 5 ). While the alloxazinic form of [LC]Li was still preferred in a nonpolar solvent ( ε : 3.04) by 0.101 eV similar to the result in vacuum condition, the isoalloxazinic form became more stable by 0.016 eV in a polar solvent ( ε : 78.4). This result implies that the choice of electrolyte strongly affects the electrochemical reaction path of tautomeric redox compounds. For the fully discharged [LC]Li 2 , the second Li prefered to be located between N1 and O2 more than other positions, which accompanied proton transfer from N1 to N10. Furthermore, the charge densities successively increased on nitrogen and oxygen atoms during two-step lithiation ( Supplementary Fig. 5 ). These results agree with the aforementioned ex situ spectroscopy results and confirm that nitrogen and oxygen atoms work as collaborative centres for the tautomerism-involving redox reaction. Molecular simplification to minimal diazabutadiene redox unit Inspired by the remarkable electrochemical activity of LC, we further tested ALX and LMZ with theoretical capacities of 250 and 327 mAh g −1 , respectively, assuming that they store two lithium atoms per molecule similar to rivoflavin and LC electrodes. The feasiblity of the electrochemical activity was first screened by computationally reducing each molecule. In the HOMO plot of the reduced ALX and LMZ, the effective delocalization of electron clouds was observed up to two electrons, suggesting that they can be utilized as redox centres for two lithium-ion storage ( Fig. 4a ). DFT calculations with actual lithium occupancies in each molecule confirmed that two lithium ions could be stored in both ALX and LMZ by undergoing similar tautomerism-accompanied redox reactions as LC ( Supplementary Figs 6 and 7 ). 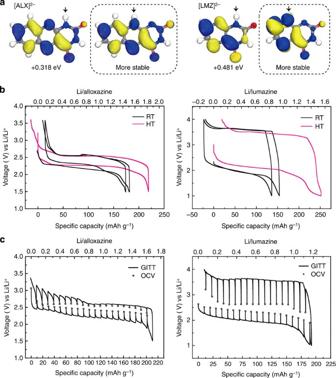Figure 4: Energy storage in ALX and LMZ. (a) HOMO plots for the doubly reduced species of ALX and LMZ. Black arrows indicate the proton that is bound to N1 or N10. (b) Capacity–voltage profiles of ALX and LMZ electrodes at room temperature (black) and 60 °C (red). (c) GITT profiles of the ALX/Li cells (left) and LMZ/Li cells (right). Figure 4: Energy storage in ALX and LMZ. ( a ) HOMO plots for the doubly reduced species of ALX and LMZ. Black arrows indicate the proton that is bound to N1 or N10. ( b ) Capacity–voltage profiles of ALX and LMZ electrodes at room temperature (black) and 60 °C (red). ( c ) GITT profiles of the ALX/Li cells (left) and LMZ/Li cells (right). Full size image We next explored the electrochemcal activity of ALX and LMZ electrodes in Li cells. As predicted by our calculations, more than one lithium ion and electron were reversibly stored in each molecule of ALX and LMZ, respectively. The ALX/Li cell showed a specific capacity of 181 mAh g −1 at 20.0 mA g −1 current density, corresponding to 1.45 Li atoms per molecule ( Fig. 4b , left). The GITT measurement with a lower current rate indicated that a capacity of 211 mAh g −1 (1.69 Li/ALX) could be reversibly delivered. Analogous to the LC electrode, the electrochemical profile could be divided into two redox steps with average OCVs of 2.52 and 2.42 V, respectively, which implied that two consecutive one-electron transfer reactions similarly occurred for ALX as well. In contrast, the LMZ electrode showed slightly different electrochemical profiles compared with LC and ALX with relatively larger polarizations ( Fig. 4b , right). At room temperature, the LMZ/Li cell delivered a reversible capacity of 154 mAh g −1 , which is equivalent to only 0.94 Li atom per molecule. The limited capability of lithium storage accompanied with the large polarization of ~1.6 V ( Supplementary Fig. 8 ) indicated that the relatively low capacity of the LMZ electrode may stem from the slow electrochemical reaction of LMZ. When we offered higher temperature (60 °C) or sufficiently low current density (intermittent current of 10.0 mA g −1 ; Fig. 4c , right) to LMZ/Li cells, the electrochemical activity of LMZ improved significantly. Note that the pteridine derivatives used in this study show reasonable thermal stability up to 220 °C ( Supplementary Fig. 9 ). The LMZ/Li cells showed specific capacities of 251 mAh g −1 (1.54 Li/LMZ) and 193 mAh g −1 (1.18 Li/LMZ) under the high-temperature cycling and GITT test, respectively. It implies that two lithium ions may be stored in LMZ, which is in agreement with our calculations, however, the lithiation kinetics were slow. The underlying reason for the slow lithiation kinetics particularly for the LMZ electrode is not fully understood yet. However, we speculate that the smaller molecular framework of LMZ compared with other molecules may induce comparatively stronger electron repulsion within the molecules when accepting two electrons. In the absence of the anellated benzo ring, the small conjugated system of LMZ is likely to show less-efficient accommodation of electrons and lithium ions at the diazabutadiene motif, thereby resulting in the large polarization. This suggests that in the molecular design of the organic electrode, the power density can be sacrificed to increase the energy density as the size of the molecule decreases. While the GITT measurement indicated that lithium insertion takes place at an average potential of 2.50 and 2.20 V in the LMZ electrode, the large polarization makes it less appealing for practical batteries. Enhanced battery performance with modified electrode design Another attractive aspect of pteridine derivative electrodes is that the electrochemical performance can be easily improved by employing a modified electrode preparation. Taking advantage of abundant electron clouds in pi orbitals of aromatic pteridines, graphitic nanocarbons can immobilize the molecules through strong pi – pi interaction, which provide the redox centres with stable anchoring and a rapid electrical path. The simple solution-based process of mixing carbon nanotubes (CNTs) and organic powder followed by vacuum filtration produced highly conductive, free-standing paper, which is directly applicable as an additive-free electrode, in which the pteridine molecules were fixed onto the surface of CNTs ( Supplementary Fig. 10 ) [14] . As a result of the hybridization, the redox molecules are reassembled from crystalline particles to nanolayers on the surfaces of CNTs ( Supplementary Fig. 11 ). We found that the hybrid electrodes exhibited dramatically improved rate capability and cyclability without changes in redox potentials ( Supplementary Fig. 12 ). The rate capabilities of the hybrid electrodes at different C rates are illustrated in Fig. 5a,b . At a current density of 220 mAh g −1 , which is equivalent to a 1C rate, the LC hybrid electrode showed a specific capacity of 215 mAh g −1 . Compared with the pristine electrodes made of powdered compounds, the charge/discharge profiles of hybrid electrodes are sloppier, which is attributable to the reduced crystallinity and particle size of the active materials, as well as to the extra capacity from CNTs (~18 mAh g −1 ; Supplementary Fig. 13 ). Even at a high current density of 10.0 A g −1 corresponding to a 45.5C rate, LC provided a specific capacity of 153 mAh g −1 , corresponding to 71.1% of the capacity at the 1C rate ( Fig. 5a ). The ALX hybrid electrode could deliver a specific capacity of 236 mAh g −1 at the 1C rate (250 mA g −1 ) and 168 mAh g −1 at the 10C rate, as shown in Fig. 5b . Moreover, the LC and ALX hybrid electrodes showed remarkable capacity retentions compared with the pristine electrodes ( Fig. 5c ; Supplementary Fig. 14 ). After 200 cycles at 1.0 and 2.0 A g −1 , the LC hybrids showed 93 and 96% capacity retention, and the ALX hybrids showed 92 and 97% capacity retention, respectively. Even after cycling up to 500 times, the LC hybrid electrodes exhibited the capacity retention above 93 and 96% at a high rate of 5.0 and 10.0 A g −1 ( Fig. 5d ), respectively. In addition, the ALX hybrid electrodes retained 93 and 91% of their initial capacity at 5.0 and 10.0 A g −1 , respectively. To the best of our knowledge, the capacity retention of 96% up to 500 cycles at 10.0 A g −1 is the best and the longest cycling performance among the organic molecule-based cathode materials reported thus far [11] , [15] , [16] , [36] . 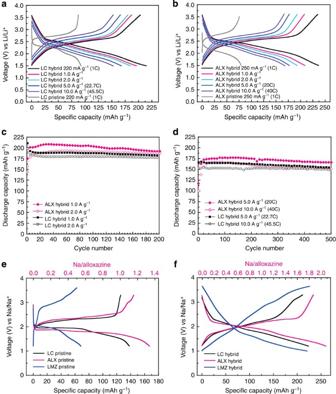Figure 5: Battery performances of modified pteridine electrodes. (a) Capacity–voltage profiles of LC-CNT hybrid electrodes (LC hybrid) at various current rates and a pristine LC electrode at a 1C rate. (b) Capacity–voltage profiles of ALX-CNT hybrid electrodes (ALX hybrid) at various current rates and a pristine ALX electrode at a 1C rate. Capacity retention of the LC hybrid and ALX hybrid (c) at 1.0 and 2.0 A g−1for 200 cycles and (d) at 5.0 and 10.0 A g−1for 500 cycles. Capacity–voltage profiles of (e) pristine pteridine derivatives at 20 mA g−1and (f) pteridine hybrid electrodes at 50 mA g−1in sodium rechargeable batteries. Figure 5: Battery performances of modified pteridine electrodes. ( a ) Capacity–voltage profiles of LC-CNT hybrid electrodes (LC hybrid) at various current rates and a pristine LC electrode at a 1C rate. ( b ) Capacity–voltage profiles of ALX-CNT hybrid electrodes (ALX hybrid) at various current rates and a pristine ALX electrode at a 1C rate. Capacity retention of the LC hybrid and ALX hybrid ( c ) at 1.0 and 2.0 A g −1 for 200 cycles and ( d ) at 5.0 and 10.0 A g −1 for 500 cycles. Capacity–voltage profiles of ( e ) pristine pteridine derivatives at 20 mA g −1 and ( f ) pteridine hybrid electrodes at 50 mA g −1 in sodium rechargeable batteries. Full size image Sodium storage in pteridine systems As the limited abundance of lithium increases the need for alternative carrier ions in rechargeable battery systems [37] , we report that pteridine-based organic electrodes are also electrochemically active to sodium. As potential cathodes in sodium rechargeable batteries, we evaluated the electrochemical reactivity of pteridine derivatives to sodium using a half cell with sodium metal. Figure 5e shows that pteridine derivatives are capable of reversibly taking up and releasing two sodium ions, representing them as versatile electrodes in rechargeable batteries. In sodium batteries, LC and ALX exhibited a specific capacity of 138 and 168 mAh g −1 , respectively, and LMZ delivered a slightly lower capacity of 70 mAh g −1 at a current density of 10.0 mA g −1 . By incorporating CNTs during electrode preparation, the deliverable capacities were significantly improved to 222, 255 and 220 mAh g −1 even at 50.0 mA g −1 for LC, ALX and LMZ, respectively ( Fig. 5f ), although the capacity could not be stably retained during repeated cycling (~50% retention after 20 cycles for all compounds). The limited cyclability could be attributable to the non-optimized Na electrolytes of the cell and the large strain of the electrode materials during the insertion of large sodium ions, which may induce the isolation of the active materials from the electrodes. While further studies are required, the sodium-organic battery system is promising for sustainable energy storage systems, since it is based on abundant sodium elements on earth and does not contain transition metals [38] , [39] , [40] . The utilization of diazabutadiene redox cycling should provide potential opportunities for sodium-organic battery systems. We described a molecular simplification strategy using tailored pteridine derivatives that contain the redox-active diazabutadiene motif of flavins to develop green and high-performance energy storage systems. For the first time, reversible tautomerism between alloxazinic and isoalloxazinic structures in pteridine derivatives during lithium-coupled electron uptake and donation was demonstrated through analyses of both ex situ characterization and DFT calculations. The pteridine-based electrode with conductive CNT scaffolds exhibited high gravimetric energy density up to 533 Wh kg −1 within a 1-h discharge, and the gravimetric energy density of 348 Wh kg −1 was demonstrated even at the high powers greater than 20 kW kg −1 . Up to 96% capacity was retained in the pteridine-based hybrid electrode after cycling 500 times at 10.0 A g −1 , which is the best and longest cycling performance at such a high rate among organic molecule-based cathode materials. Also, the utilization of diazabutadiene redox cycling in sodium-ion batteries was first proposed, while further study is required to overcome the capacity fading. The current study suggests that various unexplored redox molecules from natural energy transduction systems can provide unlimited opportunities to design sustainable electrodes with superior performances beyond the conventional electrode materials of rechargeable lithium/sodium-ion batteries. Electrochemistry Cyclic voltammograms of pteridine derivatives (0.5 mM) were captured using TBAP and LiClO 4 electrolytes (0.1 M) in DMF solution under N 2 atmosphere. A three-electrode system (Pt counter electrode, Ag/AgCl reference electrode, glassy carbon working electrode) was employed and the scan rate was 100 mV s −1 . Electrochemical profiles of LC, ALX and LMZ powder samples were measured versus a Li metal foil (Hohsen, Japan) and a Na metal cube (Sigma Aldrich, USA) in coin-type cells (CR2016). The electrodes were fabricated by mixing 40% w/w active materials, 40% w/w conductive carbon (Super P) and 20% w/w polytetrafluoroethylene (PTFE) binder for both Li- and Na-ion cells. We adjusted the total amounts of electrodes within the range of 6.0±1.0 mg per cell. The electrodes were dried overnight at 60 °C under vacuum. In the modified electrode preparation, hybrid electrodes were produced by mixing the organic compounds and single-walled CNTs in acetone using a sonicator followed by vacuum filtration. The resulting self-standing paper was directly used as an electrode without current collectors and additives for both Li- and Na-ion cells. According to the elemental analysis, the portions of active materials in the hybrid electrodes were 43, 41 and 35wt% for LC, ALX and LMZ, respectively. The average weight of the free-standing electrodes was ~1.0 mg per cell. A porous glass microfiber membrane (GF/F; Whatman, UK) was used as a separator in both the Li- and Na-ion cells. The electrolytes were 1 M LiPF 6 in tetraethylene glycol dimethyl ether (TEGDME, Techno Semichem, Korea) for Li-ion cells and 1 M NaPF 6 in diethylene glycol dimethyl ether (DEGDME) for Na-ion cells. The cells were assembled under inert atmosphere in an Ar-filled glove box. Galvanostatic measurements were performed at various constant current densities on a battery test system (Won-A, Korea). Ex situ electrode characterization For ex situ analyses, the electrodes were prepared by disassembling coin cells at different states of charge (as-prepared, half-discharged and fully discharged to 1.6 V, half-charged and fully recharged to 3.6 V) followed by rinsing the electrodes with dimethyl carbonate. To prevent exposure to air, all samples were sealed in an Ar-filled glove box. XPS measurements were conducted with a Thermo VG Scientific Sigma Probe spectrometer (UK) equipped with a microfocus monochromated X-ray source (90 W). Binding energies were referenced to the C–C bond of the C 1s region at 284.5 eV. Fourier transform infrared spectra were recorded with pellets made of active powders scraped out of the electrodes and KBr powder on an FT/IR-4200 (Jasco, Japan) at a resolution of 2 cm −1 under vacuum. For fluorescence spectroscopy, samples were immersed in degassed deionized water under a nitrogen atmosphere, resulting in solubilized active molecules. Fluorescence spectra were obtained using a V/650 spectrophotometer (Jasco) in the range of 400–600 nm. Computational details Geometry optimization and energy calculations on the molecules were conducted with spin-unrestricted DFT using the Gaussian 09 quantum chemistry package [41] based on the Becke–Lee–Yang–Parr (B3LYP) hybrid exchange-correlation functional [42] , [43] , [44] and the standard TZVP basis set [45] , [46] , [47] . The site and sequence of lithium occupation during the redox reaction were determined by comparing DFT energies of possible reduced forms of molecules bonded to one or two lithium ions. Atomic charge was calculated using Mulliken population analysis [48] . A detailed procedure and the results of DFT calculations are discussed in the Supplementary Information . The HOMO plots were generated with the cubegen utility, which was embedded in Gaussian 09 (ref. 41 ) and visualized with the Materials Studio program. How to cite this article : Hong, J. et al. Biologically inspired pteridine redox centres for rechargeable batteries. Nat. Commun. 5:5335 doi: 10.1038/ncomms6335 (2014).